Microporous metal-organic framework with potential for carbon dioxide capture at ambient conditions Carbon dioxide capture and separation are important industrial processes that allow the use of carbon dioxide for the production of a range of chemical products and materials, and to minimize the effects of carbon dioxide emission. Porous metal-organic frameworks are promising materials to achieve such separations and to replace current technologies, which use aqueous solvents to chemically absorb carbon dioxide. Here we show that a metal-organic frameworks (UTSA-16) displays high uptake (160 cm 3 cm −3 ) of CO 2 at ambient conditions, making it a potentially useful adsorbent material for post-combustion carbon dioxide capture and biogas stream purification. This has been further confirmed by simulated breakthrough experiments. The high storage capacities and selectivities of UTSA-16 for carbon dioxide capture are attributed to the optimal pore cages and the strong binding sites to carbon dioxide, which have been demonstrated by neutron diffraction studies. Carbon dioxide (CO 2 ) emissions have become one of the most serious issues and environmental concerns facing our civilization today [1] . These emissions are mainly generated from the combustion of coal, oil and natural gas, the main energy resources for our daily life, economic growth and industrial development [2] . Before we realize the cleaner alternative energy and establish the energy infrastructure for the implementation of new materials and technologies in the future, CO 2 emissions will continue to increase; it is thus very important and mandatory for us to capture and separate CO 2 to minimize their environmental impact. The state-of-the-art technology to capture CO 2 makes use of aqueous alkanolamine absorbents to chemically absorb CO 2 (ref. 3 ). This technology costs a large amount of regeneration energy, because the CO 2 can only be released at quite a high elevated temperature, owing to the strong interactions of the CO 2 with these absorbents (the typical enthalpy of absorption lies the range of −50 to −100 kJ mol −1 at 296 K and low CO 2 loadings) and the high boiling points of these alkanolamine absorbents; in fact, CO 2 captured from a post-combustion flue gas using this technology results in an energy penalty of about 30% of the output of the power plant [4] . Furthermore, this technology will also lead to some environmental issues owing to the corrosive nature of these absorbents. The emerging porous metal-organic frameworks (MOFs) are promising as the cost-effective and efficient materials for CO 2 capture and separation [5] , [6] , [7] , [8] , [9] , [10] . The regeneration energy cost to utilize these porous materials for CO 2 capture by the implementation of temperature swing adsorption, pressure swing adsorption (PSA) and vacuum swing adsorption is significantly lower than the abovementioned alkanolamine technology. More importantly, the rapid development over the past decade in this research field to target some porous MOFs for their extremely high uptake of CO 2 at high pressure [11] , [12] and to immobilize functional sites, such as open metal sites [13] , [14] , [15] , [16] , [17] , [18] , [19] , [20] , [21] , [22] , [23] , –NH 2 and –OH organic sites into the pore surfaces to enhance their interactions and thus enforce their efficient CO 2 separation selectivity have principally ensured the feasibility of porous MOFs for CO 2 capture [24] , [25] , [26] , [27] , [28] , [29] , [30] , [31] , [32] , [33] , [34] , [35] , [36] , [37] , [38] . Although porous MOFs are principally feasible for CO 2 capture, realization of some practically useful MOF materials for its implementation is still challenging. The flue gas generated from the combustion of coal in the air consists of low content of CO 2 (15–16%) and high content of N 2 , and is released at a total pressure of approximately 1 bar, although the CO 2 capture from methane in biogas streams should be realized at ambient conditions, which means that the ideal MOF materials for these CO 2 capture should be those exhibiting extraordinarily high CO 2 uptake and selectivity at near-ambient pressures. Furthermore, they should be highly stable, particularly in the small amount of moisture, and can be easily regenerated for long-term usage. For practical applications, high volumetric CO 2 adsorption capacities are even more important than gravimetric CO 2 adsorption capacities for the temperature swing adsorption, PSA and vacuum swing adsorption post-combustion CO 2 capture and separation to fully utilize the fixed-bed space and minimize the energy regeneration cost. To screen a series of porous MOFs synthesized in our own laboratory having different pore structures, surface areas and pore-surface functionalities, herein we report the performance of an adsorbent [K(H 2 O) 2 Co 3 (cit)(Hcit)] [39] (we term this MOF UTSA-16; UTSA=University of Texas at San Antonio; H 4 cit=citric acid) for efficient CO 2 capture at room temperature and 1 bar. Its potential for CO 2 capture has been further examined by simulated PSA for the breakthrough separation of CO 2 (50%)/CH 4 (50%) mixture (biogas streams) and CO 2 (15%)/N 2 (85%) flue gas mixture (post-combustion CO 2 capture), highlighting UTSA-16 as a promising material with high separation selectivity and capacity for CO 2 capture applications at ambient conditions. Neutron diffraction studies reveal that both suitable pore/cage space and the terminal water molecules have enabled their strong interactions with CO 2 molecules, and thus collaboratively enforced the high separation selectivity and capacity of this MOF material for CO 2 capture and separation at ambient conditions. Examined MOF materials The examined porous MOFs are general ones (Zn 4 O(FMA) 3 , UTSA-33a) without any specific functional sites, those with open Cu(II) sites (UTSA-20a and UTSA-34b), open Zn(II) sites (Zn 4 (OH) 2 (1,2,4-BTC) 2 and Zn 5 (BTA) 6 (TDA) 2 ) and open Yb(III) sites (Yb(BPT)), those with functional –OH sites on the pore surfaces (UTSA-15a, UTSA-25a and Cu(BDC-OH)) and one with the terminal water molecules (UTSA-16) [39] . Their structural features, pore characteristics and adsorption isotherms are shown in Supplementary Table S1 and Supplementary Figs S1 and S2 . As established by Krishna and Long [40] , the separation performance of porous materials in PSA separation of gas mixtures is strongly influenced by capacity considerations. For this reason, we systematically use volumetric CO 2 uptake capacities to characterize the performance of the reported MOF materials. As shown in Supplementary Fig. S1 , UTSA-16 takes up significantly large amount of CO 2 (160 cm 3 cm −3 ) at 296 K and 1 bar, which is at least three times higher than the rest of the porous MOFs (even some of these porous MOFs exhibit higher porosities, as shown Supplementary Table S1 ). That is really remarkable. The high CO 2 adsorption of UTSA-16 has featured it to be the second highest porous MOF for CO 2 capture and separation at 296 K and 1 bar (the best known MOF is Mg-MOF-74 (ref. 18 ) with storage capacity of 162 cm 3 cm −3 ). For comparing the separation performance of these MOFs synthesized in our group, we selected a number of MOFs for which the separation data has been reported, and for which the required isotherm data are available in the literature. The chosen MOFs are as follows: CuBTC [41] , Mg-MOF-74 (refs 15 , 17 , 42 ), Zn(bdc)(dabco) 0.5 (ref. 43 ), MIL-101 (ref. 41 ), Cu-TDPAT [44] , bio-MOF-11 (ref. 45 ), MOF-177 (ref. 17 ), ZIF-78 (ref. 28 ) and ZnMOF-74 (refs 20 , 46 , 47 ). Supplementary Table S2 provides the structural data and pore characteristics for these chosen MOFs. The measured experimental data on pure component isotherms for CO 2 , CH 4 and N 2 at 273 and 296 K in our synthesized MOFs, and those literature data of temperature-dependent single component CO 2 , CH 4 and N 2 sorption isotherms for the chosen MOFs were first converted to absolute loadings, using the Peng–Robinson equation of state for estimation of the fluid densities. Depending on the guest-host combination, the choice of the isotherm is either a 1-site Langmuir or a 2-site Langmuir, or a 2-site Langmuir–Freundlich model. The isotherm models selected along with the fit parameters are specified in Supplementary Tables S3–33 . For comparison, the absolute loading of CO 2 on UTSA-16 and the chosen MOFs at 296 K is shown in Fig. 1 , indicating that the CO 2 loading on UTSA-16 is slightly lower than Mg-MOF-74, but higher than the rest of MOFs. The loading dependence of Q st for CO 2 in different MOFs, determined using the pure component isotherm fits, is compared in Fig. 2a and Supplementary Tables S34 . 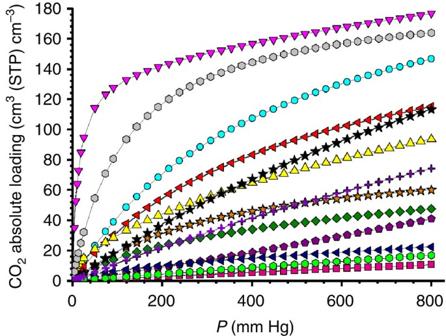Figure 1: Comparison of the absolute loading of CO2at 296 K. From top to bottom, MgMOF-74 (magenta down triangle), UTSA-16 (grey hexagon), ZnMOF-74 (cyan circle), bio-MOF-11 (red left triangle), CuBTC (black star), Cu-TDPAT (yellow up triangle), UTSA-20a (violet cross), ZIF-78 (orange star), Zn5(BTA)6(TDA)2(olive diamond), Zn(bdc)(dabco) (purple pentagon), MIL-101 (navy left triangle), Yb(BPT) (green hexagon) and MOF-177 (pink square). Figure 1: Comparison of the absolute loading of CO 2 at 296 K. From top to bottom, MgMOF-74 (magenta down triangle), UTSA-16 (grey hexagon), ZnMOF-74 (cyan circle), bio-MOF-11 (red left triangle), CuBTC (black star), Cu-TDPAT (yellow up triangle), UTSA-20a (violet cross), ZIF-78 (orange star), Zn 5 (BTA) 6 (TDA) 2 (olive diamond), Zn(bdc)(dabco) (purple pentagon), MIL-101 (navy left triangle), Yb(BPT) (green hexagon) and MOF-177 (pink square). 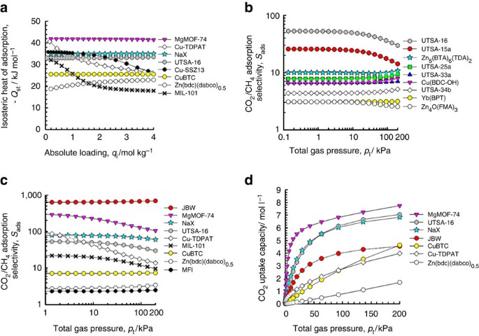Figure 2: IAST calculations for binary CO2/CH4mixtures on the MOFs. (a) Comparison of the loading dependence of the isosteric heats of pure CO2adsorption on the porous materials. (b,c) CO2/CH4adsorption selectivity for the variety of MOFs considered in this work. (d) CO2uptake volumetric capacity of some important MOFs. In these calculations, the partial pressures of CO2and CH4are taken to be equal to each other, that is,p1=p2=100 Pa. All calculations are for 296 K, using theT-dependent isotherm parameters reported inSupplementary Tables S3–S33. The calculations of theQstof Cu-TDPAT are those reported in the paper by Liet al.44 Full size image Figure 2: IAST calculations for binary CO 2 /CH 4 mixtures on the MOFs. ( a ) Comparison of the loading dependence of the isosteric heats of pure CO 2 adsorption on the porous materials. ( b , c ) CO 2 /CH 4 adsorption selectivity for the variety of MOFs considered in this work. ( d ) CO 2 uptake volumetric capacity of some important MOFs. In these calculations, the partial pressures of CO 2 and CH 4 are taken to be equal to each other, that is, p 1 = p 2 =100 Pa. All calculations are for 296 K, using the T -dependent isotherm parameters reported in Supplementary Tables S3–S33 . The calculations of the Q st of Cu-TDPAT are those reported in the paper by Li et al . [44] Full size image IAST calculations for binary CO 2 /CH 4 mixtures We compared the performance of our MOFs with several MOFs (Mg-MOF-74, Cu-TDPAT, CuBTC, MIL-101 and Zn(BDC)(DABCO) 0.5 ) for CO 2 capture and separation from CO 2 (1)/CH 4 (2) mixtures containing 50 mole% CO 2 , and maintained at isothermal conditions at 296 K and pressures up to 200 kPa. For comparison purposes, three zeolites (NaX [42] , [48] , JBW and MFI) [49] with high selectivity were also considered for analysis. Using the pure component isotherm fits, the adsorption selectivities defined by were determined using the IAST of Myers and Prausnitz [50] . The accuracy of the IAST calculations for estimation of the component loadings for several binary mixtures in a wide variety of zeolites and MOFs has been well established by comparison with the Configurational-Biast Monte Carlo simulations of mixture adsorption [49] . We proceeded further to determine the CO 2 /CH 4 adsorption selectivities for the different MOFs at 296 K. In these calculations, the partial pressures of CO 2 and CH 4 are taken to be equal to each other, that is, p 1 = p 2 . As shown in Fig. 2b,c , UTSA-16 has a higher selectivity than the other MOFs reported from our own lab and most reported MOFs in the literature, although it has a lower CO 2 /CH 4 selectivity than Mg-MOF-74. The specific orbital interactions of CO 2 molecules with the open Mg atoms accounts for the high selectivities offered by Mg-MOF-74 (refs 20 , 51 , 52 , 53 ). Among all the pore materials, JBW has the highest selectivity, followed by Mg-MOF-74, NaX and UTSA-16. For ease of comparison, Supplementary Table S35 presents the numerical data on the adsorption CO 2 /CH 4 selectivities at 200 kPa and 296 K in different MOFs. Besides separation selectivity, capacity considerations are important in determining the performance of any given adsorbents in a PSA unit. The loading of CO 2 in the adsorbed phase within the porous structures in equilibrium with a binary CO 2 /CH 4 gas mixture maintained at isothermal conditions at 296 K were determined for a range of pressures up to 200 kPa. For a total pressure of 200 kPa, the data on gravimetric uptake capacities are listed in Supplementary Table S35 . At this pressure, we note that CO 2 uptake capacity of Mg-MOF-74 is about twice as high as any other material. JBW has a low uptake capacity because of its low pore volume [54] . We will see later that JBW will have poor performance in a PSA unit. Because of the wide differences in the framework densities, the hierarchy of CO 2 uptake capacities is quite different when expressed as mol l −1 of adsorbent; the corresponding data are presented in Fig. 2d . We now note that UTSA-16 is only slightly lower than Mg-MOF-74 in terms of their volumetric uptake capacities and both of them exhibit significantly higher volumetric storage capacities than the rest of MOFs. The volumetric uptake capacity of UTSA-16 is comparable to that of the NaX zeolite. Breakthrough calculations for PSA adsorber Most commonly, the adsorption selectivity on its own is used to screen MOFs for any separation task. The performance of an MOF in a PSA unit is governed by both selectivity and capacity factors. The proper combination of both of these factors is obtained by use of breakthrough calculations [40] . 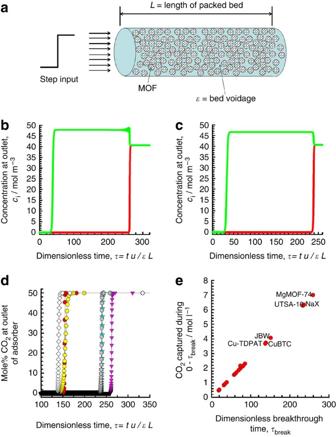Figure 3: Breakthrough calculations for PSA adsorber. (a) Schematic of a packed bed adsorber. Breakthrough characteristics of an adsorber packed with (b) Mg-MOF-74 and (c) UTSA-16 and maintained at isothermal conditions at 296 K. In these calculations, the partial pressures of CO2and CH4at the inlet is taken to bep1=p2=100 kPa. (d) Plot of the number of moles of CO2captured per litre of adsorbent material during the time interval 0–τbreakagainst the breakthrough timeτbreakfor packed bed adsorber with step-input of a 50/50 CO2/CH4mixture at 296 K and total pressures of 200 kPa. The breakthrough times,τbreak, correspond to those when the outlet gas contains 0.05 mole% CO2. The considered MOFs are MgMOF-74 (purple down triangle), NaX (cyan star), UTSA-16 (grey hexagon), JBW (red circle), CuBTC (yellow circle) and Cu-TDPAT (open diamond). (e) Plot of the number of moles of CO2captured from CO2/CH4mixture per litre of adsorbent material, during the time interval 0–τbreakagainst the breakthrough timeτbreakfor packed bed adsorber with step-input of a 50/50 CO2/CH4mixture at 296 K and total pressures of 200 kPa. The breakthrough times,τbreak, correspond to those when the outlet gas contains 0.05 mole% CO2. Figure 3a shows a schematic of a packed bed adsorber. The breakthrough calculations were performed using the following methodologies developed and described in earlier works [40] , [54] , [55] ; the breakthrough simulation methodology has been validated by direct comparison with experimental breakthrough data in the work of Bloch [56] . Figure 3b and present typical breakthrough curves for Mg-MOF-74 and UTSA-16, respectively. The x axis in Fig. 3b–d is a dimensionless time, τ , defined by dividing the actual time, t , by the characteristic time, L / u . Figure 3d shows the gas composition, expressed as mole% CO 2 in outlet gas as a function of the dimensionless time for a selection of porous adsorbent materials. On the basis of these calculations, the value of the breakthrough time, τ break , can be determined for a specified purity of CO 2 in the outlet gas stream. For an arbitrarily chosen purity of 0.05 mole% CO 2 , the data of dimensionless breakthrough times are presented in Supplementary Table S36 . It shows that Mg-MOF-74 and UTSA-16 have τ break of 259 and 234, respectively, which are significantly higher than for Cu-BTC (139), Cu-TDPAT (138), ZIF-78 (81) and rest of the MOFs. UTSA-16 has the comparable τ break with the best zeolite NaX (235). A longer τ break is desirable because the frequency of regeneration is reduced. It needs to be mentioned that although JBW zeolite has the highest CO 2 /CH 4 adsorption separation selectivity, its breakthrough time is much shorter than UTSA-16 ( Fig. 3d ). Figure 3: Breakthrough calculations for PSA adsorber. ( a ) Schematic of a packed bed adsorber. Breakthrough characteristics of an adsorber packed with ( b ) Mg-MOF-74 and ( c ) UTSA-16 and maintained at isothermal conditions at 296 K. In these calculations, the partial pressures of CO 2 and CH 4 at the inlet is taken to be p 1 = p 2 =100 kPa. ( d ) Plot of the number of moles of CO 2 captured per litre of adsorbent material during the time interval 0– τ break against the breakthrough time τ break for packed bed adsorber with step-input of a 50/50 CO 2 /CH 4 mixture at 296 K and total pressures of 200 kPa. The breakthrough times, τ break , correspond to those when the outlet gas contains 0.05 mole% CO 2 . The considered MOFs are MgMOF-74 (purple down triangle), NaX (cyan star), UTSA-16 (grey hexagon), JBW (red circle), CuBTC (yellow circle) and Cu-TDPAT (open diamond). ( e ) Plot of the number of moles of CO 2 captured from CO 2 /CH 4 mixture per litre of adsorbent material, during the time interval 0– τ break against the breakthrough time τ break for packed bed adsorber with step-input of a 50/50 CO 2 /CH 4 mixture at 296 K and total pressures of 200 kPa. The breakthrough times, τ break , correspond to those when the outlet gas contains 0.05 mole% CO 2 . Full size image The economics of a PSA unit for post-combustion CO 2 capture will be dictated primarily by the amount of CO 2 captured during the adsorption cycle, that is, during the time interval 0– τ break ; this amount can be determined from a material balance; the data on the amount adsorbed is also presented in Supplementary Table S36 . The CO 2 capture presented in Supplementary Table S36 is expressed both in mol kg −1 of adsorbent and mol l −1 of adsorbent material. The proper metric for comparing different adsorbents for use in a PSA unit is on the basis of moles captured per litre of adsorbent. This is because an existing adsorber will have a fixed volume. When considering the choice of the best MOF to replace the existing adsorbent, we should compare these on the capture capacity per litre of adsorbent. Figure 3e presents plots of the number of moles of CO 2 captured per litre of adsorbent against the breakthrough time τ break . It is remarkable to note that per litre of adsorbent material, the number of moles of CO 2 capture is almost perfectly linearly related to the dimensionless breakthrough time. This is a rational result. The breakthrough calculations for different materials were performed with the same volume of adsorber, containing identical volumes of adsorbent materials. Expressed differently, Fig. 3e demonstrates that the proper metric that determines the separation characteristics of a PSA adsorber is the dimensionless breakthrough time, τ break , which in turn depends on both selectivity and capacity metrics. From a practical point of view, the volumetric capture capacity is more relevant for screening and choosing the suitable MOFs. Apparently, UTSA-16 is a superior adsorbent for CO 2 /CH 4 separation at ambient conditions than most MOFs, other than MgMOF-74. Comparison of MOFs for CO 2 /N 2 separation We further compared the performance of UTSA-16 with several MOFs (mmen-CuBTTri, Mg-MOF-74, MOF-177, ZIF-78, Cu-TDPAT, bioMOF-11, Zn-MOF-74) for CO 2 capture from CO 2 (1)/N 2 (2) mixtures containing 15 mole% CO 2 , and maintained at isothermal conditions at 296 K, which represent conditions relevant for flue gas processing. For comparison, five representative zeolites (NaX [42] , [48] , Cu-SSZ13 [57] , H-SSZ13 [57] , JBW [49] and MFI [49] ) exhibiting high CO 2 /N 2 separation selectivity are also included. 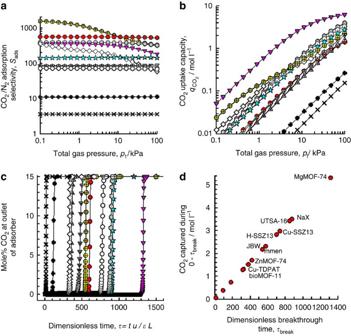Figure 4: Comparison of MOFs for CO2/N2separation. Calculations using Ideal Adsorbed Solution Theory (IAST) of Myers and Prausnitz50for (a) CO2/N2adsorption selectivity, and (b) volumetric CO2uptake capacity in equilibrium with a binary CO2/N2gas mixture maintained at isothermal conditions at 296 K. In these calculations, the partial pressures of CO2and N2are taken to bep1/p2=15/85. (c) CO2/N2mixture breakthrough characteristics in terms of mole% CO2in outlet gas as a function of the dimensionless time in an adsorber packed with different adsorbents and maintained at isothermal conditions at 296 K. In these calculations, the partial pressures of CO2and N2are taken to bep1=15 kPa andp2=85 kPa. The considered MOFs fromatocare MgMOF-74 (purple down triangle), NaX (cyan star), UTSA-16 (grey hexagon), JBW (red circle), mmen-CuBTTri (yellow plus-centered circle), Cu-SSZ13 (open circle), ZnMOF-74 (plus-centered down triangle), bio-MOF-11 (plus-centered up triangle), Cu-TDPAT (open diamond), MFI (black plus) and MOF-177 (black cross). (d) Plot of the number of moles of CO2captured from CO2/N2mixture per litre of adsorbent material, during the time interval 0–τbreakagainst the breakthrough timeτbreakfor packed bed adsorber with step-input of a 15/85 CO2/N2mixture at 296 K and total pressures of 100 kPa. The breakthrough times,τbreak, correspond to those when the outlet gas contains 0.05 mole % CO2. Figure 4a presents the IAST calculations for CO 2 /N 2 adsorption selectivity. We note that the selectivities for different MOF materials vary by about two orders of magnitude. Among the MOFs, amine-functionalized mmen-CuBTTri has the highest adsorption selectivity followed closely by UTSA-16 and Mg-MOF-74. The lowest adsorption selectivity is obtained with MOF-177 that has the most open structure of all MOF materials considered here, which is apparently not favourable for low-pressure CO 2 capture. JBW has the highest adsorption selectivity but a poor uptake capacity because of its low pore volume [54] . Figure 4: Comparison of MOFs for CO 2 /N 2 separation. Calculations using Ideal Adsorbed Solution Theory (IAST) of Myers and Prausnitz [50] for ( a ) CO 2 /N 2 adsorption selectivity, and ( b ) volumetric CO 2 uptake capacity in equilibrium with a binary CO 2 /N 2 gas mixture maintained at isothermal conditions at 296 K. In these calculations, the partial pressures of CO 2 and N 2 are taken to be p 1 / p 2 =15/85. ( c ) CO 2 /N 2 mixture breakthrough characteristics in terms of mole% CO 2 in outlet gas as a function of the dimensionless time in an adsorber packed with different adsorbents and maintained at isothermal conditions at 296 K. In these calculations, the partial pressures of CO 2 and N 2 are taken to be p 1 =15 kPa and p 2 =85 kPa. The considered MOFs from a to c are MgMOF-74 (purple down triangle), NaX (cyan star), UTSA-16 (grey hexagon), JBW (red circle), mmen-CuBTTri (yellow plus-centered circle), Cu-SSZ13 (open circle), ZnMOF-74 (plus-centered down triangle), bio-MOF-11 (plus-centered up triangle), Cu-TDPAT (open diamond), MFI (black plus) and MOF-177 (black cross). ( d ) Plot of the number of moles of CO 2 captured from CO 2 /N 2 mixture per litre of adsorbent material, during the time interval 0– τ break against the breakthrough time τ break for packed bed adsorber with step-input of a 15/85 CO 2 /N 2 mixture at 296 K and total pressures of 100 kPa. The breakthrough times, τ break , correspond to those when the outlet gas contains 0.05 mole % CO 2 . Full size image Figure 4b shows data on the CO 2 uptake capacity expressed as mol l −1 of adsorbent. The highest uptake capacity is afforded by Mg-MOF-74, and this is closely followed by UTSA-16. The lowest uptake is offered by MOF-177. The data on the selectivity and capacity for operation at a total pressure of 100 kPa are also summarized in Supplementary Table S37 . To evaluate the different adsorbents for use in a PSA unit, breakthrough calculations were performed. Figure 4c compares the breakthrough characteristics in terms of mole% CO 2 in outlet gas as a function of the dimensionless time for operation at a total pressure of 100 kPa. Supplementary Table S38 summarizes the data on dimensionless breakthrough times. The breakthrough times are a reflection of the combination of the selectivity and capacity metrics. The longest breakthrough time is obtained with Mg-MOF-74. The reason for this can be traced to a combination of high selectivities and high capacities. This is followed by NaX zeolite and UTSA-16. It is particularly noteworthy that JBW and mmenCuBTTri that exhibit extremely high selectivities have significantly shorter breakthrough times. This is because both have low uptake capacities. The shortest breakthrough time is obtained with MOF-177; ZIF-78 has only a slightly higher breakthrough time. Figure 4d presents plots of the number of moles of CO 2 captured per litre of adsorbent material, during the time interval 0– τ break against the breakthrough time τ break . We note that there is a perfect linear correlation between the amount captured per litre of adsorbent and τ break , in line with the findings of this study reported in Fig. 4d . This re-emphasizes the conclusion that the dimensionless breakthrough time is the proper metric to reflect the separation performance of any MOF in a PSA unit. Mg-MOF-74 ends up at the desirable top-right corner of Fig. 4d . It is interesting to note that Cu-TDPAT does not possess the required combination of selectivity and capacity to be a viable candidate for post-combustion CO 2 capture in PSA operations. The lowest capture capacity is with MOF-177, with ZIF-78 displaying only slightly better performance. This point is being stressed here because of the special attention given by Bae and Snurr [58] to ZIF-78 in their recent review as the best adsorbent for CO 2 capture. This further underlines the need for a proper comparison of different MOFs using the breakthrough analysis presented here. Another interesting point to note is that the amount of CO 2 captured per litre of adsorbent material follows the hierarchy Mg-MOF-74>UTSA-16≈NaX, similar to the hierarchy determined for separation of CO 2 /CH 4 mixtures; compare Figs 3e and 4d . Comparison with Cu-(bpy-1) 2 During the writing of this manuscript, the paper of Burd et al . [59] appeared online, in which the authors present the uptake data for CO 2 , CH 4 and N 2 at 296 K in Cu-(bpy-1) 2 . We scanned their experimental data presented in Fig. 2 of their paper, converted to absolute component loadings, fitted the pure component isotherms and calculated the adsorption selectivities, using IAST, of Cu-(bpy-1) 2 for separation of CO 2 /CH 4 and CO 2 /N 2 mixtures. For CO 2 /CH 4 mixtures, our IAST calculations agree very well with those reported in Fig. 3 of their paper. Supplementary Fig. S3 presents a comparison of the CO 2 /CH 4 adsorption selectivity of Cu-(bpy-1) 2 with that for the variety of MOFs considered in this work. We note that UTSA-16 has a significantly higher selectivity than Cu-(bpy-1) 2 . Supplementary Fig. S4 presents a comparison of the CO 2 /N 2 adsorption selectivity of Cu-(bpy-1) 2 with that for the variety of MOFs considered in this work. We note, once again, that UTSA-16 has a significantly higher selectivity than Cu-(bpy-1) 2 . Neutron diffraction studies The extraordinary performance of UTSA-16 for the CO 2 capture at ambient conditions has motivated us to rationalize the crucial factors to enforce the high CO 2 adsorption selectivity and capacity. To experimentally verify the preferential adsorption sites and thus to elucidate the highest density of CO 2 trapped into its pore, neutron-powder diffraction (NPD) data were collected on UTSA-16 loaded with 0.45 CO 2 per coordinated H 2 O, using the high-resolution neutron powder diffractometer (BT-1) at the NIST Center for Neutron Research. The Rietveld refinement was performed on the NPD data using the programme EXGUI, yielding the agreement factors of R wp =0.0345, R p =0.0292 and χ 2 =1.17. The Rietveld fit to the diffraction pattern is shown in Supplementary Fig. S5 . From the refinement, CO 2 is only adsorbed at one site with 0.45 CO 2 per co-ordinated H 2 O loading, that is, the total amount of CO 2 molecules obtained from the refinement is in good agreement with the target value for the CO 2 loading in the host lattice. The crystal structure of the CO 2 -loaded UTSA-16 is shown in Fig. 5 . 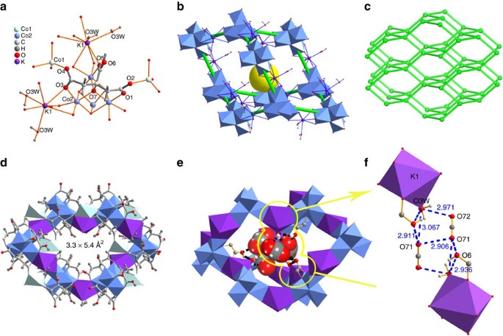Figure 5: The structure for CO2-loaded UTSA-16. (a) The coordination mode of citrate ligand. Each citrate chelates one cubic (Co(2)4O4) cluster, two Co(1) tetrahedral and two K ions. There are two water (O3w) coordinated to each K ions. (b) Each cubic (Co(2)4O4) cluster node is linked by four K polyhedral linkers to give a diamondoid cage (yellow ball of about 4.5 Å in diameter). There are four crystallographically independent O3w from 4 K polyhedral toward the cage. For clarity, Co1, C and H on citrate ligand are omitted. The linkages between the cubic clusters are present with the green sticks (not the real bond) to illustrate the framework topology. (c) The resultingdianetwork. (d) The diamondoid cage has a small widow with the dimensions of 3.3×5.4 Å2. All metal ions are present as the polyhedral with the colours same as those for the atoms ina. (e) A couple of CO2dimers are trapped within the cage; (f) The cooperative interactions between CO2molecules and the framework (O71(CO2)...O71(CO2) and O71(CO2)...O6 short contact; O72(CO2)...H-O3w, O71(CO2)...H-O3w and O3w...H-O6 hydrogen-bonding interactions). The angle between the two linear CO2molecules is of 64.93(2)°. Figure 5: The structure for CO 2 -loaded UTSA-16. ( a ) The coordination mode of citrate ligand. Each citrate chelates one cubic (Co(2) 4 O 4 ) cluster, two Co(1) tetrahedral and two K ions. There are two water (O3w) coordinated to each K ions. ( b ) Each cubic (Co(2) 4 O 4 ) cluster node is linked by four K polyhedral linkers to give a diamondoid cage (yellow ball of about 4.5 Å in diameter). There are four crystallographically independent O3w from 4 K polyhedral toward the cage. For clarity, Co1, C and H on citrate ligand are omitted. The linkages between the cubic clusters are present with the green sticks (not the real bond) to illustrate the framework topology. ( c ) The resulting dia network. ( d ) The diamondoid cage has a small widow with the dimensions of 3.3×5.4 Å 2 . All metal ions are present as the polyhedral with the colours same as those for the atoms in a . ( e ) A couple of CO 2 dimers are trapped within the cage; ( f ) The cooperative interactions between CO 2 molecules and the framework (O71(CO 2 ) ... O71(CO 2 ) and O71(CO 2 ) ... O6 short contact; O72(CO 2 ) ... H-O3w, O71(CO 2 ) ... H-O3w and O3w ... H-O6 hydrogen-bonding interactions). The angle between the two linear CO 2 molecules is of 64.93(2)°. Full size image The structure of CO 2 -loaded UTSA-16 is a three-dimensional framework in which the coordination environments and framework topology are shown in Fig. 5a–c . As shown in Fig. 5d , the pore window is about 3.3×5.4 Å 2 . The diamondoid cage of about 4.5 Å in diameter can trap two pairs of CO 2 molecules ( Fig. 5e ) through UTSA-16 K-OH 2 ···O 2 C hydrogen-bonding interactions (O3w-H···O72=2.971(1) Å, <O3w-H···O72=102.05(4)°; O3w-H···O71=3.067(1) Å, <O3w-H···O71=135.98(4)°) and O···O close contact (O71···O6=2.911(2) Å; O71···O71=2.906(1) Å), as shown in Fig. 5f . The angle between the two linear CO 2 molecules is of 64.93°. On the basis of the stoichiometric ratio 1:1 of CO 2 to coordinated water, the density and uptake capacity of trapped CO 2 will be 0.768 g cm −3 and 118 cm 3 (STP) cm −3 . The remaining uptake of 42 cm 3 (STP) cm −3 might be attributed from the empty pore space, which accounts for 26% total CO 2 uptake capacity, highlighting the crucial contribution from the interactions between the O atom of CO 2 adsorbate and the O atoms (O3w and O6) on the pore surfaces. The nearest intermolecular O···O contact between CO 2 molecules trapped in UTSA-16 is shorter than those reported in other CO 2 -loaded MOFs ( Supplementary Table S39 ). The density of the CO 2 in UTSA-16 is approximately equal to the liquid CO 2 density of 1.032 g cm −3 (ref. 60 ), estimated according to the amount of gas adsorbed and the Platon pore volume (30.2%) of the framework of 1.037 g cm −3 at 1 atm and 296 K, which is the highest ever reported on the MOFs for CO 2 capture at the same condition. The highest CO 2 density means UTSA-16 can trap CO 2 in the most efficient mode into its pore to reach saturation even at 296 K and 1 atm ( Supplementary Fig. S6 ), featuring UTSA-16 as the very promising material for the highly selective separation of CO 2 from the light gases. In summary, the uniqueness of UTSA-16 for its highly selective separation of CO 2 from the light gases is attributed to the following factors: (1) stable diamondoid network comprising of (Co 4 O 4 ) clusters and K-polyhedra linkers via face-sharing, which is supported by the infinite three-dimensional heteronuclear M-O-M connections, (2) diamondoid cage of 4.5 Å in diameter to efficiently trap two pairs of CO 2 molecules, (3) small widows of 3.3×5.4 Å 2 for its potentially high size-selective effect (the kinetic molecule sizes for CO 2 , N 2 and CH 4 are 3.30, 3.64 and 3.80 Å, respectively), and (4) four crystallographically dependent coordinated water molecules within each cavity for their hydrogen-bonding interactions with the CO 2 gas molecules. The microporous MOFs are promising materials for CO 2 capture and separation. As we can rationally design and synthesize some highly porous MOFs, which can take up significant amount of CO 2 under high pressure (a few extremely highly porous MOFs with BET surface areas over 6,000 m 2 g −1 have been constructed; The CO 2 storage capacities at room temperature and high pressure are basically proportional to the surface areas of the MOF materials) [12] , it is quite straightforward and feasible to realize MOF materials for high-pressure CO 2 capture and separation. The CO 2 storage capacities at room temperature and low pressure (1 bar; essential conditions for CO 2 capture and separation in post-combustion mixtures and biogas streams), however, are not dependent on their pore surface areas, which have been clearly demonstrated in our examined MOF materials and literatures. Such a situation poses a great challenge to synthetic materials chemists on how to target some unique porous MOF materials, for which CO 2 capture can be significantly high at ambient conditions. Ideally, we already have the resolution, that is, to immobilize specific sites such as open metal sites and –NH 2 sites to induce their strong interactions with CO 2 , and to optimize the pore/cage sizes to maximize the van der Waals interactions between the pore surfaces and CO 2 . However, only a few porous MOFs have been realized for high CO 2 capture at ambient conditions. The fact that Mg-MOF-74 takes up much more CO 2 than other M-MOF-74 (M=Ni 2+ , Co 2+ , Zn 2+ and Fe 2+ ), and some other porous MOFs with open metal sites (for example, UTSA-20a and Yb(BPT) in this report) do not necessarily exhibit high CO 2 uptake at room temperature and 1 bar, indicates that both different type of open-metal sites and MOF structures have important roles to enforce their strong interactions with CO 2 at ambient conditions. Mg-MOF-74 is very unique because of its extremely high CO 2 uptake at room temperature and 1 bar. However, because the interactions of Mg-MOF-74 with water molecules are very strong, Mg-MOF-74 is highly sensitivity to the moisture, leading to its significantly reduced CO 2 storage capacities once it is exposed to the air. UTSA-16 exhibits repeatable and reversible CO 2 sorption ( Supplementary Fig. S7 ). More importantly, the re-activated UTSA-16 from the used sample, which has been exposed in the air for 3 days, still keeps the same sorption capacities for CO 2 , indicating that UTSA-16 is not air sensitive. Such properties are apparently important for its potential industrial usage. It needs to be mentioned that the existence of the coordinated water molecules is essential for UTSA-16 to have high CO 2 capture capacity. In fact, once all the water molecules within UTSA-16 are removed at elevated temperature, the resulting anhydrous material is non-porous. Another advantage of UTSA-16 for it's CO 2 capture and separation is it's cheap cost of the raw materials, particularly the very common organic linker citric acid, which should allow us to enlarge the synthesis straightforwardly. Our accidental discovery of UTSA-16 for high CO 2 capture and separation at ambient conditions might facilitate the extensive research on porous MOF materials for CO 2 capture in the near future. Synthesis and gas adsorption All reagents and solvents employed in synthetic studies were commercially available and used as supplied without further purification. As-synthesized sample UTSA-16 was synthesized, activated accordingly to our reference procedures [39] , and confirmed by powder X-ray diffraction study and N 2 adsorption isotherms. The detailed synthetic procedures are in the following: the hydrothermal reaction of Co(OAc) 2 ·4H 2 O (0.249 g 1 mmol), C 6 H 8 O 7 ·H 2 O (0.21 g, 1 mmol), KOH (0.168 g, 3 mmol), H 2 O (2.5 ml) and C 2 H 5 OH (2.5 ml) in the molar ratio 1:1:3:139:43 is conducted in a teflon-lined 23 ml Parr acid digestion bomb. The bomb is then placed in a furnace that is heated from room temperature to 120 °C in half an hour, kept at 120 °C for 2 days, and then slowly cooled to room temperature at a rate of 4 °C h −1 . And violet prismatic samples were obtained, which were filtered, washed with ethyl ether and dried at room temperature. The sample is degassed for 24 h at 363 K and 5 μm Hg to obtain the activated UTSA-16. Overactivation at higher temperature and vacuum will lead to the collapse of the framework and non-porous material. The preparation and activation methods for other MOFs synthesized in our lab were followed our references ( Supplementary Table S1 ). CO 2 , CH 4 and N 2 adsorption isotherms for our MOFs were measured on Micromeritics ASAP 2020 Accelerated Surface Area and Porosimetry analyzer. As the centre-controlled air condition was set up at 23.0 °C, a water bath of 23.0 °C was used for gas adsorption isotherms at 296.0 K. Fits of pure component isotherms for the pore materials The measured experimental data on pure component isotherms for CO 2 , CH 4 and N 2 at 273 K and 296 K in the MOFs synthesized in our lab, and the literature data of temperature-dependent single component CO 2 , CH 4 and N 2 sorption isotherms for the chosen MOFs and the representative zeolites were first converted to absolute loadings, using the Peng–Robinson equation of state for estimation of the fluid densities. The pore volume data given in Supplementary Tables S1 and S2 were used for this purpose. Depending on the guest–host combination the choice of the isotherm is either a 1-site Langmuir, or a 2-site Langmuir, or a 2-site Langmuir–Freundlich model. The isotherm models selected along with the fit parameters are specified in Supplementary Tables S3–S33 . Isosteric heat of adsorption The isosteric heat of adsorption, Q st , defined as were determined using the pure component isotherm fits for the 11 MOFs synthesized in this study. For some guest–host combinations for which either the dual-site Langmuir or dual-site Langmuir–Freundlich fits were used, Q st is a function of the loading. The Q st values for CO 2 and CH 4 for the 11 different MOFs synthesized in this work are reported in Supplementary Table S34 . The values are for the loadings corresponding to that in equilibrium with a bulk gas pressure of 100 kPa at 296 K. The loading dependence of Q st for CO 2 in different MOFs is compared in Fig. 2a for some important MOFs that emerge in this study as promising candidates for CO 2 /CH 4 and CO 2 /N 2 separations. Breakthrough calculations for PSA adsorber The breakthrough calculations were performed using the following the methodologies developed and described in earlier works [40] , [54] , [55] . Assuming plug flow of CO 2 (1)/CH 4 (2) or CO 2 (1)/N 2 (2) gas mixture through a fixed bed maintained under isothermal conditions and negligible pressure drop, the partial pressures in the gas phase at any position and instant of time are obtained by solving the following set of partial differential equations for each of the species i in the gas mixture. In equation (3), t is the time, z is the distance along the adsorber, ρ is the framework density, is the bed voidage, and u is the superficial gas velocity. The molar loadings of the species i , q i , at any position z , and time t is determined from the IAST calculations. Details of the numerical procedures used are available in earlier works [40] , [54] , [55] . Specifically, the calculations presented here were performed taking the following parameter values: bed length, L =0.3 m; voidage of bed, =0.4; superficial gas velocity and u =0.04 m s −1 (at inlet). When comparing different materials, the fractional voidage is held constant at =0.4. This implies the volume of adsorbents remains the same. The total mass of the adsorbents used is governed by the framework density. NPD studies NPD data were collected on the high-resolution neutron powder diffractometer (BT-1) at the NIST Center for Neutron Research with a Cu(311) monochromator and using in-pile collimation of 15 min of arc, corresponding to a wavelength of 1.5403 Å. The activated UTSA-16 sample was first degassed under vacuum and transferred to a cylindrical vanadium can equipped with a capillary gas line and a packless valve, and sealed with an indium O-ring in a helium-filled glove box. The sample can was then mounted onto a sample stick, equipped with a stainless steel gas line with an additional valve for a top-loading closed-cycle helium refrigerator (CCR). Targeted amount of CO 2 , that is 0.45 CO 2 per coordinated H 2 O, was then loaded into the UTSA-16 sample at room temperature. The sample was slowly cooled to 210 K at which point the CO 2 was completely adsorbed. Once the system was equilibrated at 210 K, the sample was further cooled to 4 K before the NPD measurement. No evidence of solid CO 2 was observed on the structural refinement, indicating all CO 2 was adsorbed into the UTSA-16. NPD data were analysed using the Rietveld refinement method with the programme EXPGUI. The CO 2 molecule was treated as a linear rigid body with a C–O bond length of 1.15 Å. Atomic positional and rotational coordinates, a thermal factor and occupancy were refined for the CO 2 site. The final refinements on all the parameters, including atomic positions, thermal factors, occupancies for both framework and adsorbed CO 2 molecules, and lattice parameters yielded very good agreement factors of R wp =0.0345, R p =0.0292 and χ 2 =1.17 ( Supplementary Fig. S5 ). Also, the total amount of CO 2 molecules obtained from the refinement is in very good agreement with the target values for the CO 2 loading in the UTSA-16 host lattice. This is another indication of the high quality of the refined structure. Accession codes: The X-ray crystallographic coordinates for structures reported in this Article have been deposited at the Cambridge Crystallographic Data Centre (CCDC), under deposition number CCDC 869399. These data can be obtained free of charge from The Cambridge Crystallographic Data Centre via http:\\www.ccdc.cam.ac.uk/data_request/cif . A summary table of crystal data is also given in the Supporting Information. How to cite this article: Xiang, S. et al . Microporous metal-organic framework with potential for carbon dioxide capture at ambient conditions. Nat. Commun. 3:954 doi: 10.1038/ncomms1956 (2012).